MiR-9 promotes microglial activation by targeting MCPIP1 Microglia participate in innate inflammatory responses within the central nervous system. The highly conserved microRNA-9 (miR-9) plays critical roles in neurogenesis as well as axonal extension. Its role in microglial inflammatory responses, however, remains poorly understood. Here we identify a unique role of miR-9 in mediating the microglial inflammatory response via distinct signalling pathways. MiR-9-mediated regulation of cellular activation involved downregulated expression of the target protein, monocyte chemotactic protein-induced protein 1 (MCPIP1) that is crucial for controlling inflammation. Results indicate that miR-9-mediated cellular activation involved signalling via the NF-κB pathway, but not the β-catenin pathway. Microglia, cells of the myeloid lineage in the central nervous system (CNS), play an important role in immune surveillance and are known to be actively involved in various neurologic pathologies. Under normal CNS homeostasis, microglia manifest a ramified phenotype with highly branched, motile cell processes [1] , [2] . In response to pathological stimuli, these cells undergo phenotypic changes, elicit inflammatory responses and migrate towards the toxic stimuli. Paradoxically, these cells while crucial for host defence, can also contribute to neuropathology if the inflammatory response remains unchecked [3] . The role of the activated microglia in neuroinflammation is intrinsic in various neurodegenerative disorders such as multiple sclerosis [4] , [5] , Parkinson’s Disease [6] , Alzheimer’s disease [7] , NeuroAIDS [8] , stroke and traumatic brain injury [9] . Understanding the regulation of microglial activation is thus critical to comprehend the inflammatory processes extant in the CNS pathology. In keeping with the emerging interest in molecular mechanisms controlling the magnitude of microglia-mediated inflammatory responses in the CNS, a new and exciting aspect of gene regulation has gained attention in recent years with the discovery of mammalian microRNAs (miRNAs) [10] , [11] , [12] . MiRNAs are small, evolutionarily conserved noncoding RNAs that are derived from much larger primary transcripts. Recent studies have demonstrated that miRNAs expressed by immune cells can target proteins regulating inflammation, and consequently affect the magnitude of the immune response [13] . MiRNAs are becoming increasingly recognized as important regulators of cell functions including glial activation [13] , [14] , [15] , [16] , [17] , [18] , [19] . While microRNA-9 (miR-9) has a well-established role in proliferation/migration of neuronal precursors [20] , [21] , [22] and axon extension/branching [23] , its role in mediating microglial activation remains poorly understood. In recent years, monocyte chemotactic protein-induced protein 1 (MCPIP1) was reported to control inflammation [24] , [25] . It was shown that MCPIP1 was a negative regulator of macrophage activation [25] and that this anti-inflammatory role was mediated via the inhibition of expression of key proinflammatory cytokines. MCPIP1 was also induced by various inflammatory stimuli including MCP-1 and lipopolysaccharide (LPS) in a variety of cell types [26] , [27] , [28] , [29] . Regulation of MCPIP1 expression by noncoding RNAs, however, has never been explored. To identify the miRNAs targeting evolutionary conserved sequences in the MCPIP1 gene (ZC3H12A), computational algorithm such as TargetScan was employed and it was found that miR-9 that is conserved among the vertebrates was predicted to target MCPIP1. In the present study, we report that miR-9 downregulates MCPIP1 expression and induces the activation of microglia. MiR-9 promotes microglial activation in in vitro and in vivo We first demonstrated the expression of miR-9 in primary rat microglia using fluorescent in situ hybridization (FISH; Fig. 1a ). To explore the role of miR-9 in microglial activation, primary mouse microglia were transduced with the lentivirus expressing miR-9 precursor ( Supplementary Fig. 13 ) and assessed for upregulation of the activation marker CD11b by flow cytometry analysis using anti-mouse CD11b antibody ( Fig. 1b ). MiR-9 mediated activation skewed the cells to an M1 phenotype with the upregulation of inducible nitric oxide synthase and interleukin-1β (IL-1β) and a concomitant downregulation of the M2a phenotype (arginase I, transforming growth factor-β and Mrc). There was no change in the M2c phenotype ( Supplementary Fig. 1a ) in primary rat microglia. These findings were also validated at the protein level using western blots for representative proteins of the microglial phenotypes ( Supplementary Fig. 1b ). The effect of miR-9 on microglial activation was further confirmed using Luminex and Nitrite assays demonstrating increased expression of the proinflammatory cytokines (IL-1β, tumour-necrosis factor-α (TNF-α), IL-6 & MCP-1; Fig. 1c ) and NO ( Fig. 1d ) in primary rat microglia. Reciprocally, transducing cells with the miRNA inhibitor, miR-9-5p-locker but not miR-9-3p-locker, had the opposing effects ( Fig. 1e,f ; Supplementary Fig. 1c ). The extent of miR-9 overexpression and knockdown was assessed by Northern blot assay ( Supplementary Fig. 2 ). Our findings demonstrated that miR-9 was critical for the activation of microglia. It must be stated that one of the unavoidable caveats of the in vitro study involving primary microglia is their inherent ability to become activated during culturing conditions. We therefore sought to validate in vivo the role of miR-9 by microinjecting lentivirus miR-9 into the substantia nigra (SNr) of CX3CR1-GFP mice, which resulted in an increased microglial activation compared with the miR-control injected group ( Fig. 1g ). 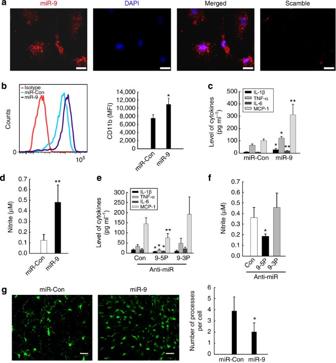Figure 1: miR-9 regulates microglial activation. (a)In situhybridization of mature miR-9 in primary rat microglia. Scale bar, 5μm. (b) Primary mouse microglia infected with miR-control or miR-9 lentivirus were assessed for CD11b expression by flow cytometry using anti-mouse CD11b antibody. All the data are indicated as mean±s.d. of four individual experiments. *P<0.05 versus miR-control group using Student’st-test. MiR-9-mediated effects on the expression of cytokines (c) and NO production (d) in primary rat microglia. Anti-miR-9-5p/9-3p mediated effects on cytokine expression (e) and NO production (f) in primary rat microglia. All the data are indicated as mean±s.d. of four individual experiments. *P<0.05; **P<0.01 versus miR-control group using Student’st-test analysis. (g) MiR-9 induced microglial activationin vivoin CX3CR1-GFP mice. Representative images of GFP+microglia (left panel) and the average number of processes per cell (right panel). Scale bar, 25 μm. All the data are indicated as mean±s.d. of four individual experiments. *P<0.05 versus miR-control group using Student’st-test. Figure 1: miR-9 regulates microglial activation. ( a ) In situ hybridization of mature miR-9 in primary rat microglia. Scale bar, 5μm. ( b ) Primary mouse microglia infected with miR-control or miR-9 lentivirus were assessed for CD11b expression by flow cytometry using anti-mouse CD11b antibody. All the data are indicated as mean±s.d. of four individual experiments. * P <0.05 versus miR-control group using Student’s t -test. MiR-9-mediated effects on the expression of cytokines ( c ) and NO production ( d ) in primary rat microglia. Anti-miR-9-5p/9-3p mediated effects on cytokine expression ( e ) and NO production ( f ) in primary rat microglia. All the data are indicated as mean±s.d. of four individual experiments. * P <0.05; ** P <0.01 versus miR-control group using Student’s t -test analysis. ( g ) MiR-9 induced microglial activation in vivo in CX3CR1-GFP mice. Representative images of GFP + microglia (left panel) and the average number of processes per cell (right panel). Scale bar, 25 μm. All the data are indicated as mean±s.d. of four individual experiments. * P <0.05 versus miR-control group using Student’s t -test. Full size image MiR-9 regulates MCPIP1 expression in microglia Having determined the role of miR-9 in microglial activation, we then sought to investigate the mechanism(s) underlying this effect. The next step was to predict the target of miR-9 using the TargetScan algorithm. MCPIP1, a CCCH zinc-finger ribonuclease (ZC3H12A) that has a conserved miR-9 binding site within its 3′-untranslated region (UTR) in most species, was identified as the putative target of miR-9 ( Fig. 2a ). MCPIP1 is a novel protein that plays a fundamental role in immune regulation [29] , [30] . Intriguingly, co-transfecting miR-9 overexpressing vector and pmiR-GLO plasmid with the MCPIP1 wild-type 3′-UTR resulted in downregulation of luciferase activity, with amelioration of this effect in BV-2 cells transfected with mutated MCPIP1 3′-UTR ( Fig. 2b ). In addition, the inhibition of endogenous miR-9 expression in cells transduced with anti-miR-9 resulted in an increased luciferase activity ( Fig. 2c ). In line with this finding, miR-9 regulated the expression of both MCPIP1 mRNA ( Fig. 2d ) and protein ( Fig. 2e ) in primary rat microglia. To further confirm whether the effect of miR-9 on MCPIP1 was a direct one, primary microglia were co-transfected with miR-9 in the presence of either a target protector oligo (TP-MCPIP1) that specifically protected the miR-9 binding site on the endogenous MCPIP 3′-UTR or a scramble target protector oligo. As shown in Fig. 2f , in the presence of a target protector oligo specific for miR-9 binding site, miR-9 failed to downregulate the expression of MCPIP1, a phenotype that was similar to cells transfected with the anti-miR-9 ( Fig. 2e ). 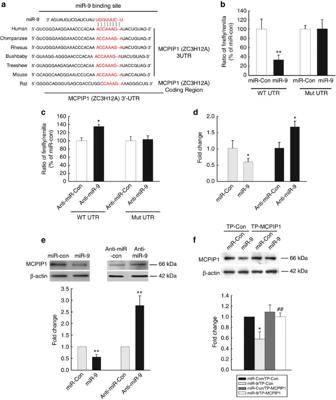Figure 2: MiR-9 regulates MCPIP1 expression in microglia. (a) Putative miR-9 binding sites in MCPIP1 gene-ZC3H12A. The potential complementary residues are shown in red. Relative luciferase activity of WT/3′UTR mutant constructs of MCPIP co-transfected with miR-control/miR-9 (b); or anti-miR-control/anti-miR-9 (c) in BV-2 cells. (d,e) Quantitative reverse transcriptase–PCR analysis of MCPIP mRNA (d) and protein (e) in primary rat microglia following transduction of cells with miR-9/anti-miR-9 constructs. All the data are indicated as mean±s.d. of four independent experiments. *P<0.05, **P<0.01 versus microglial transfected with miR-control or anti-miR-control group by Student’st-test. (f) Western blot of MCPIP1 in lysates of primary microglia co-transfected with miR-9/miR-control in the presence of either TP-MCPIP1 or scrambled oligo. Representative immunoblots (upper panel) and the densitometric analysis (lower panel) of MCPIP1/β-actin from four separate experiments. All the data are indicated as mean±s.d. of four independent experiments. *P<0.05 versus microglial transfected with miR-control and TP-control group;##P<0.01 versus microglial transfected with miR-9 and TP-control group using one-way analysis of variance followed by Holm–Sidak test. Figure 2: MiR-9 regulates MCPIP1 expression in microglia. ( a ) Putative miR-9 binding sites in MCPIP1 gene-ZC3H12A. The potential complementary residues are shown in red. Relative luciferase activity of WT/3′UTR mutant constructs of MCPIP co-transfected with miR-control/miR-9 ( b ); or anti-miR-control/anti-miR-9 ( c ) in BV-2 cells. ( d , e ) Quantitative reverse transcriptase–PCR analysis of MCPIP mRNA ( d ) and protein ( e ) in primary rat microglia following transduction of cells with miR-9/anti-miR-9 constructs. All the data are indicated as mean±s.d. of four independent experiments. * P <0.05, ** P <0.01 versus microglial transfected with miR-control or anti-miR-control group by Student’s t -test. ( f ) Western blot of MCPIP1 in lysates of primary microglia co-transfected with miR-9/miR-control in the presence of either TP-MCPIP1 or scrambled oligo. Representative immunoblots (upper panel) and the densitometric analysis (lower panel) of MCPIP1/β-actin from four separate experiments. All the data are indicated as mean±s.d. of four independent experiments. * P <0.05 versus microglial transfected with miR-control and TP-control group; ## P <0.01 versus microglial transfected with miR-9 and TP-control group using one-way analysis of variance followed by Holm–Sidak test. Full size image MCPIP1 as a functional target of miR-9 To determine whether miR-9-mediated functional effects depend specifically on MCPIP1 suppression, an expression construct encoding the entire MCPIP1 coding sequence but lacking the 3′UTR, yielding an mRNA resistant to miRNA-mediated suppression, was generated. In primary rat microglia transfected with the MCPIP1 construct lacking the UTRs (MCPIP1-Δ3′UTR), and therefore not targeted by miR-9, there was a failure of miR-9 to induce inflammatory cytokines associated with microglial activation ( Fig. 3a ) as well as the dominant M1 phenotype ( Supplementary Fig. 3 ). Consistent with this finding, transfection of primary microglia with the TP-MCPIP1 specific for miR-9 binding site resulted in amelioration of miR-9 mediated induction of inflammatory cytokines ( Fig. 3b ). 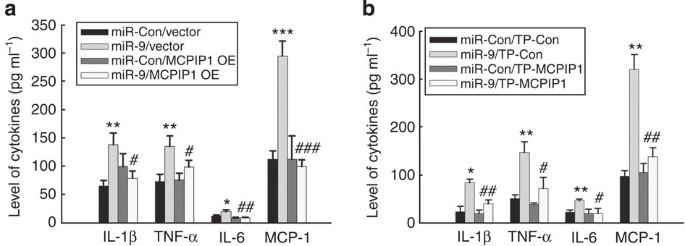Figure 3: MCPIP1 is the target of miR-9. (a) MCPIP1 Δ3′UTR overexpression rescued miR-9-mediated expression of cytokines in primary rat microglia. (b) Microglia were co-transfected with either miR-9/miR-control and TP-MCPIP1/Scramble oligo and assessed for cytokines in the supernatant by Luminex assay. All the data are indicated as mean±s.d. of four independent experiments. Presence of TP-MCPIP1 resulted in abrogation of miR-9-mediated induction of cytokines. *P<0.05, **P<0.01, ***P<0.001 versus microglial transfected with miR-control and vector/TP-control group;#P<0.05,##P<0.01,###P<0.001 versus microglial transfected with miR-9 and vector/TP-control group using one-way analysis of variance followed by Holm–Sidak test. Figure 3: MCPIP1 is the target of miR-9. ( a ) MCPIP1 Δ3′UTR overexpression rescued miR-9-mediated expression of cytokines in primary rat microglia. ( b ) Microglia were co-transfected with either miR-9/miR-control and TP-MCPIP1/Scramble oligo and assessed for cytokines in the supernatant by Luminex assay. All the data are indicated as mean±s.d. of four independent experiments. Presence of TP-MCPIP1 resulted in abrogation of miR-9-mediated induction of cytokines. * P <0.05, ** P <0.01, *** P <0.001 versus microglial transfected with miR-control and vector/TP-control group; # P <0.05, ## P <0.01, ### P <0.001 versus microglial transfected with miR-9 and vector/TP-control group using one-way analysis of variance followed by Holm–Sidak test. Full size image Involvement of NF-κB in miR-9-mediated microglial activation The next step was to determine the intracellular signalling pathways involved in miR-9-induced microglial activation. The effect of miR-9 on activation of NF-κB, AP-1 and STAT-1 was examined. BV-2 cells were transiently co-transfected with luciferase reporter constructs NF-κB-TK-Luc, AP-1-TK-Luc, or GAS-TK-luc and miR-9. In the presence of miR-9, there was an increased activation of NF-κB but not AP-1 or STAT-1 ( Fig. 4a ), and this effect was ameliorated in cells overexpressing MCPIP1 ( Fig. 4b ). Since miR-9 is known to target E-cadherin/β-catenin [31] , we next sought to examine whether overexpression with MCPIP1-Δ3′UTR could abrogate this effect. Primary rat microglia transfected with miR-9 exhibited increased the activity of β-catenin ( Fig. 4c ) and overexpression of MCPIP1 abrogated this effect ( Fig. 4d ). Further validation of miR-9-mediated nuclear translocation of NF-κB and β-catenin was demonstrated by western blot analysis ( Fig. 4e ). Reciprocally, co-transfection of primary microglia with the miR-9 construct and the TP-MCPIP1 oligo resulted in failure of miR-9 to induce activation of NF-κB and β-catenin ( Fig. 4f ). To further confirm the role of NF-κB and β-catenin as miR-9 downstream target genes, primary rat microglia were transduced with anti-miR-9-5p followed by stimulation with LPS and assessed for nuclear translocation of NF-κB ( Fig. 4g ) and β-catenin ( Fig. 4h ). As shown in Supplementary Fig. 4 , cells transduced with anti miR-9-5p, failed to exhibit LPS-mediated nuclear translocation of NF-κB and β-catenin, thereby underpinning their role as miR-9 downstream target genes. 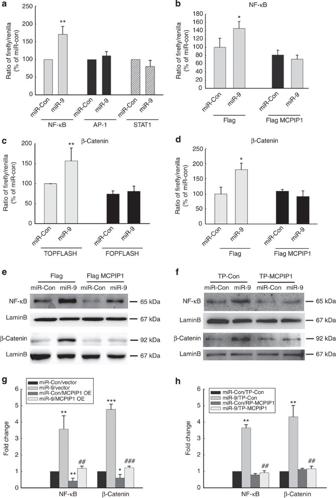Figure 4: MiR-9-mediated activation of NF-κB and β-catenin involves suppression of MCPIP1. (a) BV-2 cells transfected with NF-κB-TK-Luc, AP-1-TK-Luc or GAS-TK-Luc constructs were cotransfected with miR-9 for 24 h followed by reporter gene activity analysis using Luciferase assay. (b) MCPIP1 Δ3′UTR overexpression inhibited NF-κB activation. (c) BV-2 cells transfected with Topflash or Fopflash constructs were co-transfected with miR-9 for 24 h followed by reporter gene activity analysis using Luciferase assay. (d) MCPIP1 Δ3′UTR overexpression inhibited activation β-catenin. All the data are indicated as mean±s.d. of four individual experiments. *P<0.05, **P<0.01 versus microglial transfected with miR-control using Student’st-test. (e) Transfection of microglia with MCPIP1 Δ3′UTR construct resulted in inhibition of miR-9 mediated nuclear translocation of NF-κB and β-catenin. (f) Transfection of microglia with TP-MCPIP1 oligo resulted in inhibition of miR-9-mediated nuclear translocation of NF-κB and β-catenin. (gandh) Densitometric analysis of NFκB and beta catenin from four separate experiments. All the data are indicated as mean±s.d. of four individual experiments. *P<0.05, **P<0.01, ***P<0.001 versus microglial transfected with miR-control and vector group;##P<0.01,###P<0.001 versus microglial transfected with miR-9 and vector group using one-way analysis of variance followed by Holm–Sidak test. Figure 4: MiR-9-mediated activation of NF-κB and β-catenin involves suppression of MCPIP1. ( a ) BV-2 cells transfected with NF-κB-TK-Luc, AP-1-TK-Luc or GAS-TK-Luc constructs were cotransfected with miR-9 for 24 h followed by reporter gene activity analysis using Luciferase assay. ( b ) MCPIP1 Δ3′UTR overexpression inhibited NF-κB activation. ( c ) BV-2 cells transfected with Topflash or Fopflash constructs were co-transfected with miR-9 for 24 h followed by reporter gene activity analysis using Luciferase assay. ( d ) MCPIP1 Δ3′UTR overexpression inhibited activation β-catenin. All the data are indicated as mean±s.d. of four individual experiments. * P <0.05, ** P <0.01 versus microglial transfected with miR-control using Student’s t -test. ( e ) Transfection of microglia with MCPIP1 Δ3′UTR construct resulted in inhibition of miR-9 mediated nuclear translocation of NF-κB and β-catenin. ( f ) Transfection of microglia with TP-MCPIP1 oligo resulted in inhibition of miR-9-mediated nuclear translocation of NF-κB and β-catenin. ( g and h ) Densitometric analysis of NFκB and beta catenin from four separate experiments. All the data are indicated as mean±s.d. of four individual experiments. * P <0.05, ** P <0.01, *** P <0.001 versus microglial transfected with miR-control and vector group; ## P <0.01, ### P <0.001 versus microglial transfected with miR-9 and vector group using one-way analysis of variance followed by Holm–Sidak test. Full size image We next validated the role of downstream transcription factors (NF-κB versus β-catenin) in miR-9-mediated microglial activation in the presence or absence of LPS stimulation. As shown in Fig. 5a , pretreatment of primary rat microglia with Ikk-2 inhibitor SC514 (5 μM) significantly decreased miR-9-mediated induction of proinflammatory cytokines. Intriguingly, miR-9 potentiated the LPS-mediated activation of microglial cells and, this effect was dampened in cells pretreated with the Ikk-2 inhibitor ( Fig. 5b ). This was further confirmed by the fact that transfection of primary rat microglia with mutant IkB resulted in amelioration of miR-9-mediated induction of proinflammatory cytokines ( Fig. 5c ). In contrast, knock down of β-catenin failed to exert significant effect on miR-9-mediated induction of proinflammatory cytokines ( Fig. 5d ). Taken together, these data implied that MCPIP1/NF-κB, but not the MCPIP1/β-catenin pathway was involved in miR-9-mediated activation of microglia. 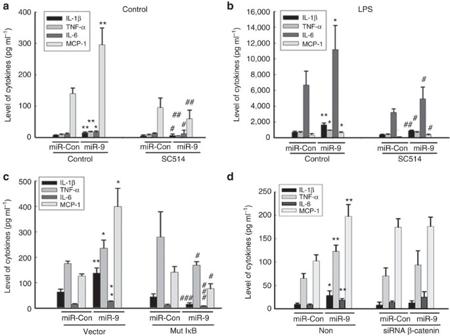Figure 5: NF-κB but not the β-catenin pathway plays a role in miR-9-mediated activation of microglia. (a,b) Primary rat microglia were transduced with miR-control or miR-9 lentivirus for 4 days and treated with Ikk-2 inhibitor-SC514 (5 μM) for 12 h. Supernatant fluids were collected and assayed by Luminex Assay for production of cytokines. All the data are indicated as mean±s.d. of four independent experiments. *P<0.05, **P<0.01 versus microglial transfected with miR-Con group;#P<0.05,##P<0.01 versus microglia transfected with miR-9 group using one-way analysis of variance (ANOVA) followed by Holm–Sidak test. (c,d) NF-κB but not β-catenin was involved in miR-9-induced microglial activation. Non: nonsense short interfering RNAs. All the data are indicated as mean±s.d. of four individual experiments. *P<0.05, **P<0.01 versus microglial transfected with miR-control and vector group;#P<0.05,###P<0.001 versus microglia transfected with miR-9 and vector group using one-way ANOVA followed by Holm–Sidak test. Figure 5: NF-κB but not the β-catenin pathway plays a role in miR-9-mediated activation of microglia. ( a , b ) Primary rat microglia were transduced with miR-control or miR-9 lentivirus for 4 days and treated with Ikk-2 inhibitor-SC514 (5 μM) for 12 h. Supernatant fluids were collected and assayed by Luminex Assay for production of cytokines. All the data are indicated as mean±s.d. of four independent experiments. * P <0.05, ** P <0.01 versus microglial transfected with miR-Con group; # P <0.05, ## P <0.01 versus microglia transfected with miR-9 group using one-way analysis of variance (ANOVA) followed by Holm–Sidak test. ( c , d ) NF-κB but not β-catenin was involved in miR-9-induced microglial activation. Non: nonsense short interfering RNAs. All the data are indicated as mean±s.d. of four individual experiments. * P <0.05, ** P <0.01 versus microglial transfected with miR-control and vector group; # P <0.05, ### P <0.001 versus microglia transfected with miR-9 and vector group using one-way ANOVA followed by Holm–Sidak test. Full size image Kinetics of LPS-mediated regulation of miR-9 and MCPIP1 The next step was to determine whether LPS mediated its effects via induction of miR-9 and also to assess the kinetics of the LPS response. Primary rat microglial cells exposed to LPS resulted in a biphasic response leading to early but significant and transient repression of miR-9 at 1 h ( Fig. 6a ), with a concomitant upregulation of MCPIP1. This was followed by a sustained and significant upregulation of miR-9 at 24 h ( Fig. 6b ). LPS-mediated regulation of miR-9 and MCPIP1 was further validated in primary rat microglial cells using Northern blotting ( Fig. 6c ), FISH ( Fig. 6d ) and immunoblot analyses, respectively ( Fig. 6e ). 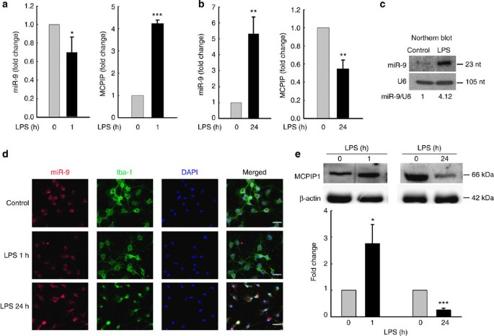Figure 6: LPS-mediated regulation of miR-9 and MCPIP1in vitro. Effect of 1 h (a) or 24 h (b) LPS stimulation (100 ng ml−1) on expression of miR-9 and MCPIP1 RNA in primary rat microglia. (c) LPS induced miR-9 expression by Northern blot in primary rat microglia (nt: nucleotides). (d) FISH of mature miR-9 in primary rat microglia treated with LPS for 1 h or 24 h. Scale bar, 5 μm. (e) Western blotting analysis of MCPIP1 expression in primary rat microglia treated with LPS for 1 or 24 h. Representative immunoblots (upper panel) and the densitometric analysis (lower panel) of MCPIP1/β-actin from four separate experiments. All the data are indicated as mean±s.d. of four independent experiments. *P<0.05, **P<0.01, ***P<0.001 versus control group using Student’st-test. Figure 6: LPS-mediated regulation of miR-9 and MCPIP1 in vitro. Effect of 1 h ( a ) or 24 h ( b ) LPS stimulation (100 ng ml −1 ) on expression of miR-9 and MCPIP1 RNA in primary rat microglia. ( c ) LPS induced miR-9 expression by Northern blot in primary rat microglia (nt: nucleotides). ( d ) FISH of mature miR-9 in primary rat microglia treated with LPS for 1 h or 24 h. Scale bar, 5 μm. ( e ) Western blotting analysis of MCPIP1 expression in primary rat microglia treated with LPS for 1 or 24 h. Representative immunoblots (upper panel) and the densitometric analysis (lower panel) of MCPIP1/β-actin from four separate experiments. All the data are indicated as mean±s.d. of four independent experiments. * P <0.05, ** P <0.01, *** P <0.001 versus control group using Student’s t -test. Full size image LPS-induced microglial activation involves miR-9/MCPIP1 axis To further assess whether miR-9 could further potentiate microglial activation induced by LPS, cells were exposed to LPS in the presence of miR-9 and assessed for proinflammatory cytokines. As shown in Fig. 7a,b , miR-9 potentiated the LPS-mediated induction of cytokines (TNF-α, IL-1β, IL-6, and MCP-1 and NO). Interestingly, and as expected, LPS-induced induction of cytokines and NO was ameliorated in cells transfected with the miR-9 inhibitor, miR-9 5P, but not 3P ( Fig. 7c,d ). Further validation of these findings was carried out in cells transfected with the TP-MCPIP1 oligo and exposed to LPS. As shown in Fig. 7e , the LPS-mediated activation of microglia was dampened in cells transfected with the target protector oligo specific for miR-9 binding site (TP-MCPIP1) compared with cells transfected with the scrambled oligo. Reciprocally, cells transfected with the miR-9 precursor demonstrated potentiation of the LPS-mediated activation of NF-κB/β-catenin pathways ( Fig. 7f,g ). Since LPS mediates translocation of NF-κB into the nucleus and since the promoter of miR-9-1 has a binding site for NF-κB [17] , we next sought to determine whether miR-9 mediated potentiation of LPS-induced microglial activation was regulated via a feedback loop between NF-κB p65 and miR-9 in primary rat microglia. Pharmacological blocking of NF-κB in microglial cells resulted in reduced ability of LPS to induce miR-9 ( Supplementary Fig. 5a ). Though NF-κB is a known downstream target of miR-9 (ref. 17 ), expression of p65 remained unaltered in the presence of miR-9 ( Supplementary Fig. 5b ). 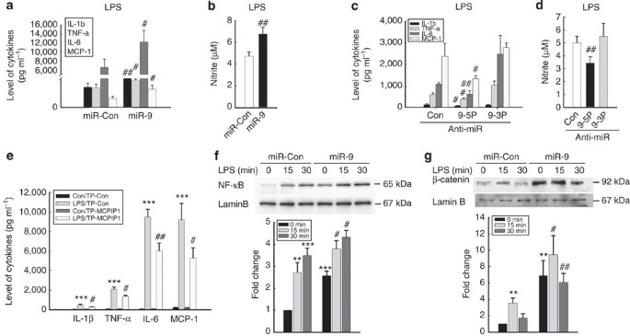Figure 7: Effect of miR-9 inhibitor on LPS-induced microglial activationin vitro. (a,b) miR-9 potentiated LPS-induced expression of cytokines (a) and NO (b) in primary rat microglia. (c,d) inhibition of miR-9 resulted in dampened expression of LPS-mediated induction of cytokines (c) and NO (d) in primary rat microglia. All the data are indicated as mean±s.d. of four independent experiments.#P<0.05,##P<0.01 versus microglial transfected with miR-control or anti-miR-control in LPS-treated group using Student’st-test analysis. (e) Transfection of TP-MCPIP1 dampened LPS-mediated induction of cytokines. All the data are indicated as mean±s.d. of four independent experiments. ***P<0.001 versus microglial transfected with TP-control in control group;#P<0.05,##P<0.01 versus microglial transfected with TP-control in the LPS group using one-way analysis of variance (ANOVA) followed by Holm–Sidak test. (f,g) MiR-9 potentiates LPS-mediated nuclear translocation of NF-κB (f) and β-catenin (g) in primary rat microglia. Representative immunoblots (upper panel) and the densitometric analysis (lower panel) of NF-κB or β-catenin/Lamin B from four separate experiments. All the data are indicated as mean±s.d. of four independent experiments. **P<0.01, ***P<0.001 versus miR-control group at 0 min;#P<0.05,##P<0.01 versus miR-control group at 15 or 30 min, respectively. This analysis was done using one-way ANOVA followed by Holm–Sidak test. Figure 7: Effect of miR-9 inhibitor on LPS-induced microglial activation in vitro. ( a , b ) miR-9 potentiated LPS-induced expression of cytokines ( a ) and NO ( b ) in primary rat microglia. ( c , d ) inhibition of miR-9 resulted in dampened expression of LPS-mediated induction of cytokines ( c ) and NO ( d ) in primary rat microglia. All the data are indicated as mean±s.d. of four independent experiments. # P <0.05, ## P <0.01 versus microglial transfected with miR-control or anti-miR-control in LPS-treated group using Student’s t -test analysis. ( e ) Transfection of TP-MCPIP1 dampened LPS-mediated induction of cytokines. All the data are indicated as mean±s.d. of four independent experiments. *** P <0.001 versus microglial transfected with TP-control in control group; # P <0.05, ## P <0.01 versus microglial transfected with TP-control in the LPS group using one-way analysis of variance (ANOVA) followed by Holm–Sidak test. ( f , g ) MiR-9 potentiates LPS-mediated nuclear translocation of NF-κB ( f ) and β-catenin ( g ) in primary rat microglia. Representative immunoblots (upper panel) and the densitometric analysis (lower panel) of NF-κB or β-catenin/Lamin B from four separate experiments. All the data are indicated as mean±s.d. of four independent experiments. ** P <0.01, *** P <0.001 versus miR-control group at 0 min; # P <0.05, ## P <0.01 versus miR-control group at 15 or 30 min, respectively. This analysis was done using one-way ANOVA followed by Holm–Sidak test. Full size image Since microglial activation is a common defining feature in various neurodegenerative diseases such as Parkinson’s disease and HAND, we also ascertained whether stimuli other than LPS such as the neurotoxins, HIV Tat or MPP + could also induce miR-9 and downregulate the expression of MCPIP1. As shown in Supplementary Figs 6,7 , both Tat and MPP + induced the expression of miR-9 and downregulated the expression of MCPIP in primary rat microglia. In concordance with these findings, Tat and MPP + also upregulated expression of proinflammatory cytokines, which was ameliorated in cells transduced with lentivirus expressing anti-miR-9 ( Supplementary Figs 6,7 ). Anti-miR-9 inhibited microglial activation in vivo To investigate the role of miR-9 in the LPS-mediated microglial activation in vivo , C57/BL6 mice were microinjected with either the control GFP lentivirus or the GFP-lentivirus-anti-miR-9 5P in the SNr and monitored for microglial activation in response to LPS. It was however, important first to determine the efficacy of GFP-lentivirus-anti-miR-9 5P transduction in vivo . As shown in Supplementary Fig. 8 , GFP expression was largely restricted within the SNr. Two weeks following lentivirus injections, mice were administered LPS daily for 4 days followed by assessment of Iba-1-positive cells in the SNr. As shown in Fig. 8a and as expected, GFP-lentivirus-microinjected mice exhibited increased microglial activation in the presence of LPS as evidenced by increased Iba-1-positive cells compared with saline-injected animals. Intriguingly, LPS-mediated increase in microglial activation was ameliorated in mice pre-treated with GFP-lentivirus-anti-miR-9 5P ( Fig. 8a ). 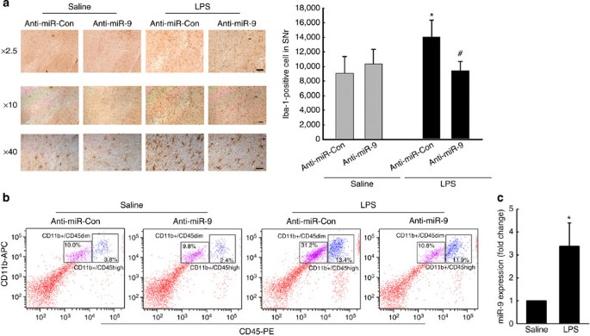Figure 8: Effect of miR-9 inhibitor on LPS-induced microglial activationin vivo. (a) Effect of anti-miR-9 on microgliosis induced by LPS in the SNr. Representative immunostained image for Iba-1 in SNr of mice injected with saline/LPS. Scale bar, 200 μm (upper panel); 100 μm (middle panel); 50 μm (lower panel). Stereology of Iba-1-positive microglia in SNr. All the data are indicated as mean±s.d.N=4 animals per group. *P<0.05 versus anti-miR group treated with saline,#P<0.05 versus anti-miR-control treated with LPS using one-way analysis of variance followed by Holm–Sidak test. (b) Effect of anti-miR-9 on the CD11b+/CD45 dim population of microglia isolated from mouse brain by Percoll gradient method and assessed by flow cytometric analysis. (c) Effect of LPS on the expression of miR-9 in microglia isolated by Percoll gradient method. Mice were injected with LPS (1 mg kg−1, i.p.) for 5 days. Total RNA isolated from microglia was subjected to real-time PCR analysis using primer sets specific for mature miR-9. All the data are indicated as mean±s.d.N=10 animals per group. *P<0.05 versus saline group using Student’st-test. Figure 8: Effect of miR-9 inhibitor on LPS-induced microglial activation in vivo. ( a ) Effect of anti-miR-9 on microgliosis induced by LPS in the SNr. Representative immunostained image for Iba-1 in SNr of mice injected with saline/LPS. Scale bar, 200 μm (upper panel); 100 μm (middle panel); 50 μm (lower panel). Stereology of Iba-1-positive microglia in SNr. All the data are indicated as mean±s.d. N =4 animals per group. * P <0.05 versus anti-miR group treated with saline, # P <0.05 versus anti-miR-control treated with LPS using one-way analysis of variance followed by Holm–Sidak test. ( b ) Effect of anti-miR-9 on the CD11b+/CD45 dim population of microglia isolated from mouse brain by Percoll gradient method and assessed by flow cytometric analysis. ( c ) Effect of LPS on the expression of miR-9 in microglia isolated by Percoll gradient method. Mice were injected with LPS (1 mg kg −1 , i.p.) for 5 days. Total RNA isolated from microglia was subjected to real-time PCR analysis using primer sets specific for mature miR-9. All the data are indicated as mean±s.d. N =10 animals per group. * P <0.05 versus saline group using Student’s t -test. Full size image Further analysis of microglia in the healthy and LPS-treated brain was performed by injecting mice bilaterally with either anti miR-control or anti-miR-9 in the SNr followed by LPS injection (ip) 2 weeks later. Five days following LPS injection microglia were isolated by Percoll gradient method and assessed by flow cytometry (CD11b+/CD45dim population). As shown in Fig. 8b , anti-miR-9 treatment resulted in decreased percentage of CD11b+/CD45dim population in the presence of LPS. The expression of miR-9 in microglia was further confirmed by the fact that LPS treatment increased miR-9 expression in sorted CD11b+/CD45dim cell population ( Fig. 8c ). Similar findings were also obtained in mice injected bilaterally with anti-miR-control or anti-miR-9 in the hippocampus ( Supplementary Fig. 9 ). These findings thus underpin the role of miR-9 in regulating the LPS-mediated microglial activation in vivo . Our study provides new insights into the role of miR-9 in regulating microglial activation via the common suppression of MCPIP1 and the distinct downstream activation of NF-κB, but not the β-catenin pathway. Modulation of miR-9/MCPIP1 can be envisioned as a therapeutic intervention for dampening microglial activation in inflammatory neurodegenerative conditions. MicroRNAs (miRs) have emerged as key regulators of the post-transcriptional control of gene expression. Previous reviews have elegantly described the pathways by which mature miRs are produced from their respective pri-miRs via nuclear cleavage and cytoplamic processing [32] . Mature miRs can mediate regulation of gene expression at the post transcriptional level by binding to either the specific sites in the 3′UTR of target mRNAs or in the coding regions of their target mRNAs, resulting in degradation or translational block, depending on the complementarity between the miRNAs and their binding sites [33] , [34] . MiR-9, a highly conserved microRNA, is expressed predominantly in the CNS of the developing embryo [35] exhibiting a pro-differentiation function [20] , [21] , [36] , [37] . MiR-9 is encoded by three distinct genomic loci miR-9-1,9-2 and 9-3 that give rise to mature miR-9 species with identical sequences. A recent study has implicated the role of mature miR-9 in controlling the stability of Hes1 mRNA and as an important player in the Hes1 ultradian oscillations [38] . MiR-9 is known to promote proliferation of neuronal progenitors by targeting stathimin, which increases microtubule instability [20] . Recent study has also reported the miR-9-mediated regulation of axonal extension and branching via targeting Map1b in mouse cortical neurons [23] . In addition to its involvement in neurogenesis, miR-9 expression also plays a role in gastric adenocarcinoma [39] . While most cells of the CNS express miR-9, a recent study indicates the lack of miR-9 activity in murine microglia under basal conditions [40] . In agreement with the findings of Akerblom et al ., our study also demonstrated no expression of miR-9 RNA in microglial cells in brain sections from control mice, however, following LPS injection, there was induction of mature miR-9 in Iba-1 positive microglia ( Supplementary Fig. 10 ). Lending credence to LPS-mediated induction of miR-9 is the finding by Bazzoni et. al . [17] , demonstrating upregulated expression of miR-9 in LPS-exposed monocytes. Consistent with this finding [17] , our study also demonstrated that exposure to LPS resulted in induced expression of pre-miR-9-1 at 6 and 12 h (2.55- and 3.85-fold), respectively ( Supplementary Fig. 11 ). There was no change in pre-miR-9-2/3 following LPS treatment. On the basis of this, the focus of our study was on the mature miR-9. Our findings for the first time demonstrate that LPS induced the expression of miR-9 in primary cultured microglia and also regulated microglial activation, both in vitro and in vivo in response to inflammatory stimuli. One possible explanation for the expression of miR-9 in untreated, cultured microglial primary cells and cell lines could be attributed to the inherent ability of these cells to become activated during cultured conditions. Taken together, our findings implicate miR-9 as a regulator of microglial activation via its suppression of the target anti-inflammatory gene MCPIP1. In pathological events such as brain inflammation, when miR-9 is upregulated, treatment with anti-miR-9 may have a beneficial effect by dampening microglial activation, thus leading to reduction of neuroinflammation. Indeed, we observed that microinjecting anti-miR-9 into the CNS resulted in deactivation and suppression of LPS-induced microglial activation. Another novel finding of this study was that MCPIP1, a novel anti-inflammatory molecule was a target of miR-9-mediated microglial activation, and these findings were confirmed in primary microglia inhibited for miR-9 activity. Briefly, knocking down of miR-9 activity via the miR-9 inhibitor or MCPIP1-target protector oligo approaches, resulted in failure of miR-9 to activate the microglia, thereby underpinning MCPIP1 as a downstream target of miR-9 mediated induction of inflammatory cytokines. These data lend credence to previous reports indicating the involvement of MCPIP1 signalling in regulating inflammatory responses via its functioning as an RNase to promote the degradation of inflammatory mRNAs such as IL-6 and IL-1β [27] and owing to its ability to function as a deubiquitinase that negatively regulates JNK and NF-κB signalling by targeting TNF receptor-associated factors [29] . In addition, elegant studies by Liang et al . [30] have also demonstrated that MCPIP1 can negatively regulate inflammatory responses as evidenced by the fact that there is increased microglial activation in MCPIP1 KO compared with the WT mice. In this study, MCPIP1 deficiency resulted in increased infarct size following ischaemic stroke [30] . Consistent with this study, our findings also suggest the role of MCPIP1 as an anti-inflammatory factor. While Liang et al . [30] observed an increased expression of MCPIP1 that was time dependent following exposure to LPS, our findings indicated a biphasic response to LPS. This discrepancy could be attributed to the strain and concentration of LPS and the conditions used in the two studies. In our study, lower concentration of LPS (10 ng ml −1 ) demonstrated a sustained increase in the expression of MCPIP1 ( Supplementary Fig. 12 ). Our findings suggested that transduction of primary microglia with miR-9 resulted in the upregulation of microglial activation markers CD11b and proinflammatory cytokines/chemokines (IL-1β, TNF-α, IL-6 and MCP-1). Intriguingly, miR-9 further potentiated LPS-induced microglial activation as evidenced by increased cytokine production. Reciprocally, inhibition of miR-9 activity via either the anti-miR-9 or the target protector oligo of MCPIP1 resulted in a dampened inflammatory response in the presence of LPS. These findings further underscore the role of miR-9/MCPIP1 axis in mediating LPS-induced generation of inflammatory cytokines. It must be noted that miR-9 was not the only pathway of LPS-mediated activation of microglia since blocking this signalling pathway did not fully abrogate the cytokine response. A possible explanation for this could be that activation of various other signalling pathways such as the TLRs could be functional in the presence of LPS. Another interesting finding of this study was that diverse activation stimuli such as HIV Tat or MPP + also mediated microglial activation via the miR-9/MCPIP1 axis thereby underscoring the role of this pathway as a common mechanism of neuroinflammation involving microglia. Using both pharmacological and genetic approaches, we demonstrated that NF-κB activation was involved in miR-9-mediated microglia activation since Ikk-2 inhibitor and transfection of microglia with mutant IkB ameliorated miR-9-mediated microglial activation. Our results are in agreement with previous reports that NF-κB activation was involved in microglial activation. Another interesting finding herein was the observation that inhibition of NF-κB resulted in failure of LPS to induce miR-9 expression. It can thus be postulated that there was a positive feedback loop between NF-κB activation and miR-9 expression since the pre-miR-9-1 promoter has a NF-κB binding site [17] . MCPIP1 is known to exert its action by inhibition of activation of NF-κB [29] . However, whether miR-9 regulates NF-κB p65 activation is unclear though NF-κB1 (p50/105) was a direct target of miR-9 (ref. 17 ). Herein we report that transduction of microglial cells with miR-9 resulted in the downregulation of MCPIP1 levels and nuclear translocation of NF-κB leading to microglial activation. These findings were also validated in vivo wherein a genetic approach using the lenti-anti-miR-9 was employed. Microinjection of lenti-anti-miR-9 into the hippocampus/SNr of mice followed by LPS injection, resulted in restoration of microglial activation thus validating the role of miR-9 in microglial activation. In summary, miR-9 plays a crucial role in microglial activation via suppression of MCPIP1 expression and subsequent downstream activation of NF-κB but not the β-catenin pathway. MiR-9/MCPIP1 axis thus mediates a regulatory pathway critical for eliciting innate immune responses in microglia. Specific blocking of the miR-9 could be considered as a potential therapeutic target for treating neuroinflammatory conditions involving microgliosis. Reagents The miR-9 overexpression has-miR-9-1 and miR-control and miR-9 inhibitor hsa-miR-9-5p-locker/hsa-miR-9-3p-locker and miR-locker-control plasmids and lentiviruses were purchased from Biosettia (San Diego). HIV-1 Tat1-72 was ordered from the UK College of Medicine, Lexington, KY. LPS ( Escherichia coli 055:B5), MPP + and Ikk-2 inhibitor-SC514 were purchased from Sigma Chemicals. Animals C57BL/6N mice (male, 6–8 weeks) were purchased from Charles River Laboratories, Inc. (Wilmington, MA). CX3CR1-GFP homozygous mice were obtained from the Jackson Laboratory (Bar Harbour, Maine) and function by targeted deletion of CX3CR1 and GFP reporter insertion. These mice are known to exhibit a rapid microglial response injury as shown by Davalos et al . [1] , [41] in response to ATP. All the animals were housed under conditions of constant temperature and humidity on a 12-h light, 12-h dark cycle, with lights on at 0700, h. Food and water were available ad libitum . Animals were deeply anaesthetized by overdose of isoflurane followed by pneumothorax before perfusion. All animal procedures were performed according to the protocols approved by the Institutional Animal Care and Use Committee of the University of Nebraska Medical Center. Cell cultures Primary microglia cells were obtained from 1 to 3-day-old C57BL/6N or Sprague–Dawley newborn pups from Charles River Laboratories, Inc.. After digestion and dissociation of the dissected brain cortices in Hank’s buffered salt solution supplemented with trypsin (1 mg ml −1 ), mixed glial cultures were prepared by resuspending the cell suspension in Dulbecco’s Modified Eagle’s Medium, supplemented with 10% heated inactivated fetal bovine serum and 10 μg ml −1 gentamicin. Cells were plated at 20 × 10 6 cells per flask density onto 75 cm 2 cell culture flasks. The cell medium was replaced each 5 days and, after the first medium change, M-CSF (0.25 ng ml −1 , macrophage colony-stimulating factor; PeproTech, Rocky Hill, NJ) was added to the flasks to promote microglial proliferation. After achieving 90% confluency mixed glial cultures were subjected to shaking at 37 °C at 220 g for 2 h, to promote microglia detachment from the flasks. The cell medium, containing the released microglia cells, was collected from each flask and centrifuged at 100 g for 5 min to collect cells and plated cell culture plates. BV-2 immortalized cells (a kind gift from Dr Sanjay Maggirwar, University of Rochester, Medical Center, Rochester, NY) were grown and routinely maintained in Dulbecco’s Modified Eagle’s Medium (4.5 g l −1 glucose; 2% fetal bovine serum; 50 mg ml −1 gentamycin) and incubated at 37 °C and 5% CO 2 . BV-2 cells were used up to passage 20. Both primary rat and mouse microglial cells were used to examine the role of miR-9 in microglial activation in vitro study. For in vivo assessment of microglial activation, primary mouse microglial cells were used. Only for the luciferase study, BV-2 cell line was used to examine the regulation of miR-9 on the transcription factors. Flow cytometry Primary mouse microglia were assayed for surface antigens by flow cytometry according to a previous report [42] . Briefly, Fc receptors were blocked with anti-mouse CD16/CD32 antibody (1:100, eBioscience). Microglial cells were stained with Alexa Fluor 488 Rat anti-mouse isotope IgG or CD11b (1:100, BD Pharmingen). LSR II (BD Biosciences) was used for fluorescence acquisition and data were analysed with FACSDiva software (BD Biosciences). For each antibody, gating was determined based on the appropriate negative isotope stained controls. Cytokine and chemokine analysis by Luminex Expression of cytokines/chemokines in supernatants collected from treated and untreated microglia was measured using MilliplexTM MAP kit (Rat Cytokine/Chemokine Magnetic Bead Panel) from Millipore as per the manufacturer’s instructions. Briefly, this is a bead-based suspension array using the Luminex MAP technology in which fluorescent-coded beads have cytokine capture antibodies on the bead surface to bind the proteins. Detailed information about the Nitrite assay can be found in Supplementary Information online . Nitrite assay Nitrite levels, a stable end product resulting from the reaction of NO with molecular oxygen, were determined in rat primary microglia by adding 50 μl of cell culture medium with 50 μl of Griess reagent (0.1% naphtyletylenediamine dihydrochloride, 1% sulphanilamide, 2.5% phosphoric acid, all from Sigma) in a 96-well plate. The absorbance at 550 nm was measured by Synergy Mx fluorescence plate reader (Bio-Tek Instruments) and nitrite concentrations were calculated using a standard curve with sodium nitrite (NaNO 2 , Sigma, level of sensitivity, 0.4 μM). Luciferase activity assays The 804 bp human MCPIP1 3′UTR containing the putative miR-9 target site was PCR amplified from human genomic DNA by using the forward 5′-ctcgctagcctcgagtctaggctgcctgtggctggcaagggcagcacccc-3′ and reverse 5′-gcctgcaggtcgactctagagaaagggctcacaatgattgtactttattg-3′ primers and the DNA fragment was cloned into the XhoI and XbaI sites on the 3′ end of the luc2 gene on the pmirGLO vector. For pmirGLO-MCPIP1 3′UTR-miR-9-target-mutant vector, the miR-9 target site (accaaag) within the MCPIP1 3′UTR was changed to ctttgtt by PCR mutagenesis with primers MCPIP1-miR-9T-F, 5′-gtcgggaaggaaacccacaactttgttatactgtaggattggttctggcccatgcag-3′ and MCPIP1-miR-9T-R, 5′-cagaaccaatcctacagtataacaaagttgtgggtttccttcccgacttgaatcctc-3′. Briefly, the BV-2 cells were transfected with miR-9 overexpression pLV-(hsa-miR-9-1) vector and the target plasmid pmirGLO-MCPIP1-3′UTR or pmirGLO-MCPIP1 3′UTR-miR-9-target-mutant in a molar ratio 50:1. The miRNA control pLV-(miR-control) plasmid was used as a negative control. The luciferase activity was determined 24 h post transfection and the reporter assay was followed the manufacturer’s protocol (Promega). Renilla luciferase activity was normalized to firefly luciferase and expressed as a percentage of the control ( n >3, performed in five wells each time). Oligos and plasmid transfection The LNA control (Scramble sequence:TAACACGTCTATACGCCCA; catalogue number480001-00) and custom-designed MCPIP1-Target Protector (TP-MCPIP1; sequence:TGGTATCTTTGGTTTGAG) were purchased from Exiqon (Woburn, MA). TP-MCPIP1 oligo selectively protects MCPIP from being targeted by miR-9, without affecting endogenous levels of miR-9 or its interaction with other mRNA targets. Microglia were transfected with 20 nmol l −1 short interfering RNAs specific for β-catenin (GAACAACGCCAGCGACAUU) were obtained from Thermo Scientific Dharmacon RNAi Technologies (Accell SMART Pool). Flag/Flag-MCPIP1, Vector/mutant IkB plasmids were transected using the SiIMPORTERTM (Millipore, Temecula, CS) according to the manufacturer’s protocol. The knockdown and transfect efficiency of short interfering RNA was determined 2 days post transfection by reverse transcriptase–PCR and western blot analysis, respectively. Western blotting Treated cells were lysed using the Mammalian Cell Lysis kit (Sigma-Aldrich). Equal amounts of the proteins were electrophoresed in a sodium dodecyl sulphate-polyacrylamide gel (12%) under reducing conditions followed by transfer to polyvinylidene fluoride membranes. The blots were blocked with 5% non-fat dry milk in PBS. The western blots were then probed with antibodies recognizing the MCPIP1 (1:1,000, Santa Cruz), β-actin (1:1,000, Sigma-Aldrich) p65 NF-κB (1:200, Cell Signalling), β-catenin (1:200, Cell Signalling), Lamin B (1:1,000, Santa Cruz) The secondary antibodies were horseradish peroxidase-conjugated to goat anti mouse/rabbit IgG (1:5,000) as described previously [43] . Full blots can be found in Supplementary Fig. 14 . Real-time PCR For quantitative analysis of mRNA expression, comparative real-time PCR was performed with the use of the SYBR Green PCR Master Mix (Applied Biosystems). The sequences for the amplification of rat MCPIP1 were: 5′-TGCCTATCACAGACCAGCAC-3′ (forward) and 5′-TGTCATTGGACACCACCACTC-3′ (reverse). The primer sequences for the amplification of GAPDH were as follows: 5′-GCCAAAAGGGTCATCATCTC-3′ (forward); 5′-GGCATGGACTGTGGTCATGAG-3′ (reverse). For the analysis of miR-9, total RNA was isolated from cells as described above. Comparative real-time PCR was performed using the Taqman Universal PCR Master Mix (Applied Biosystems). Specific primers and probes for mature miR-9 and snRNA RNU6B were obtained from Applied Biosystems. The primer sequences for the amplification of different miR-9 were as follows: mouse miR-9-1: 5′-GGTCCTGGATCC CATCTTTT-3′ (forward) and 5′-GCGCAGTGTATGGGGTTATT-3′ (reverse); mouse miR-9-2: 5′-AAGCTTAAACGCGGCAAGTA-3′ (forward) and 5′-TCGGTGACCTTGAAGGAGTT-3′ (reverse); mouse miR-9-3: 5′-GGAGTCCGTGTGTCTGTGTG-3′ (forward) and 5′-GCTTTATGA CGGCTCTGTGG-3′ (reverse). All reactions were run in triplicate. The amount of miR-9 was obtained by normalizing to snRNA RNU6B and relative to control as previously reported [44] . In situ hybridization and immunostaining Primary rat microglia (d12 in vitro ) or mouse brain sections were fixed and were prehybridized in hybridization buffer (50% formamide, 10 mM Tris-HCl, pH 8.0, 200 μg ml −1 yeast tRNA, 1 × Denhardt’s solution, 600 mM NaCl, 0.25% SDS, 1 mM EDTA, 10% Dextran sulphate) at a concentration of 9 pM for the commercially available digoxigenin-labelled miR-9 probe (Exiqon). LNA-modified miR-9, labelled at both the 5′ and 3′ ends with digoxigenin (Exiqon), were diluted to a final concentration of 2 pM in hybridization buffer, heated to 65 °C for 5 min and separately hybridized to the sections at 37 °C overnight. The slides were then washed twice in hybridization buffer (without probe) at 37 °C, followed by washing three times in 2 × SSC and twice in 0.2 × SSC at 42 °C. They were then blocked with 1% bovine serum albumin, 3% normal goat serum in 1 × PBS for 1 h at room temperature and incubated with anti-digoxigenin conjugated with horseradish peroxidase (1:100, Roche Diagnostics, Mannheim, Germany) and anti-Iba-1 (1:250, Dako) antibodies overnight at 4 °C. The slides were washed twice with PBS and incubated with Alexa Fluor 488 goat anti-rabbit IgG (1:400, Invitrogen, Carlsbad, CA) antibody for 1 h at room temperature. This was followed by two PBS washes and signal amplification (for the in situ , now labelled with horseradish peroxidase) using TSA Cy5 kit (PerkinElmer, Waltham, MA) according to the manufacturer’s protocol. The slides were mounted in Prolong gold anti-fade reagent with DAPI (Invitrogen). The specificity of the miR-9 signal in FISH experiments was confirmed when compared with a scrambled control. Unlike the miR-9, the scramble probe showed no signal in microglia. Northern blots Total RNA was extracted from primary rat microglia treated with LPS for 24 h using Trizol reagent (Invitrogen) and run on a 15% Tris/Borate/EDTA (90 mM Tris/64.6 mM boric acid/2.5 mM EDTA (pH8.3)) Urea gel (Invitrogen) and transferred to a Nytran nylon transfer membrane (Ambion, Austin, TX). The membranes were cross linked and prehybridized for at least 1h with Ultra-Hyb solution (Ambion), followed by hybridization to the LNA DIG-probe for miRNA-9 (Exiqon, Vedbaek, Denmark) or the snRNA RNU6B probe according to the manufacturer’s instructions. Transduction of primary mouse microglia with miR-9 lentivirus Primary mouse microglia were transduced with miR-Control, miR-9 lentivirus with multiplicity of infection of 100, followed by gentle swirling, incubation and replacement of fresh feed medium. The transduction efficiency was determined by detecting red fluorescent protein-positive microglia at 4 days post transduction ( Supplementary Fig. 13 ). MiR-9-induced microglial activation in vivo MiR-control or miR-9 lentivirus were microinjected into SNr in CX3CR1-GFP mice (1 μl of 10 9 viral genomes per μl) using the microinjection parameters (coordinates 2.8 mm behind the bregma, 1.7 mm lateral from the sagittal midline at a depth of 4.5 mm to skull surface). Two week later, mice were perfused and sectioned followed by assessment of number of processes for GFP + microglia from four mice per group. Anti-miR-9 ameliorated microglial activation in vivo Eight-week-old C57BL/6N mice were divided into four groups of 20 mice with each group ( n =5; male) treated with either: (1) Saline+anti-miR-control lentivirus; (2) Saline+anti-miR-9 lentivirus; (3) LPS+anti-miR-control lentivirus; (4) LPS+anti-miR-9 lentivirus. The lentiviruses were microinjected into the SNr of mice (1 μl of 10 9 viral genomes per μl) using the microinjection parameters (coordinates 2.8 mm behind the bregma, 1.7 mm lateral from the sagittal midline at a depth of 4.5 mm to skull surface). Another set of animals were microinjected with lentiviruses into hippocampus of mice (1 μl of 10 9 viral genomes per μl) using the microinjection parameters (coordinates 2.06 mm behind the bregma, ±1.5 mm lateral from the sagittal midline at a depth of 1.7 mm to skull surface). To reduce the volume of inoculation and increase the precision, a 10-μl Hamilton syringe with a 33G needle was utilized for intra-SNr/hippocampus injections as described. Two weeks later, mice were injected with LPS (1 mg kg −1 , i.p.) for 5 days. To evaluate the effect of miR-9-5p-locker on microglial activation-induced by LPS, groups of 20 mice were divided as described above, perfused and sections followed by Iba-1 staining for the assessment of microglial activation. Mouse microglia isolation Groups of mice were microinjected bilaterally either with miR-control or anti-miR-9 followed by LPS injection (described above). Five days post LPS injection, microglia were isolated from whole brain homogenates by Percoll gradient centrifugation according the previous reports [45] , [46] with slight modifications. Briefly, the brains were homogenized in PBS (pH 7.4) by passing through a 70-μm nylon cell strainer. Resulting homogenates were centrifuged at 600 g for 6 min. Supernatants were removed and cell pellets were resuspended in 70% isotonicPercoll (GE-healthcare, Uppsala, Sweden) at room temperature. A discontinuous Percoll density gradient was layered as follows: 70, 50, 35 and 0% isotonic Percoll. The gradient was centrifuged for 20 min at 2,000 g and microglia were collected from the interphase between the 70 and 50% Percoll layers. Cells were washed and then resuspended in sterile PBS followed by Flow cytometry analysis by gating the myeloid cells for the CD11b + /CD45dim population. Immunostaining and image analysis For Iba-1 immunostaining, sections encompassing the entire midbrain were sectioned at 12 μm on a cryostat. Slides were fixed with 4% paraformaldehyde for 45 min at room temperature followed by permeabilization with 0.3% Triton X-100 in PBS followed by incubation with H 2 O 2 for 10 min. Sections were incubated with a blocking buffer containing 10% NGS in PBS for 1 h at room temperature followed by addition of rabbit anti-Iba-1 (1:250; Wako) antibody and incubated overnight at 4 °C. Next day, sections were washed followed by incubation with biotinylated goat anti-rabbit immunoglobulin G (1:200) in immunoblocking buffer at RT for 1 h and incubated with an avidin-biotin-peroxidase kit for 1 h. Horseradish peroxidase reaction product was visualized with enhanced DAB peroxidase substrate kit. Every sixth section from each mouse was used to quantify Iba-1-positive cells in the midbrain and hippocampus. The immunostaining signals were quantitatively analysed using the Optical Fractionator method with Microbrightfield Stereo-Investigator software (Stereo Investigator software, Microbrightfield, VT, USA). The total number of Iba-1 microglia in entire area of SNpc was counted from four or five samples per group. Statistical analysis Statistical analysis was performed using Student’s t -test or one-way analysis of variance followed by Holm–Sidak test (SigmaPlot 11.0). The appropriate test was clarified in the figure legends. Results were judged statistically significant if P <0.05 by analysis of variance. How to cite this article: Yao, H. et al . MiR-9 promotes microglial activation by targeting MCPIP1. Nat. Commun. 5:4386 doi: 10.1038/ncomms5386 (2014).